The evolutionary origins of ritualized acoustic signals in caterpillars Animal communication signals can be highly elaborate, and researchers have long sought explanations for their evolutionary origins. For example, how did signals such as the tail-fan display of a peacock, a firefly flash or a wolf howl evolve? Animal communication theory holds that many signals evolved from non-signalling behaviours through the process of ritualization. Empirical evidence for ritualization is limited, as it is necessary to examine living relatives with varying degrees of signal evolution within a phylogenetic framework. We examine the origins of vibratory territorial signals in caterpillars using comparative and molecular phylogenetic methods. We show that a highly ritualized vibratory signal—anal scraping—originated from a locomotory behaviour—walking. Furthermore, comparative behavioural analysis supports the hypothesis that ritualized vibratory signals derive from physical fighting behaviours. Thus, contestants signal their opponents to avoid the cost of fighting. Our study provides experimental evidence for the origins of a complex communication signal, through the process of ritualization. Evolutionary origins of animal communication signals have been a major preoccupation of biologists since the time of Darwin. Many displays are thought to have evolved through the process of ritualization, whereby activities not associated with communication, such as locomotory movements, breathing or body secretions, are co-opted to create new communication signals [1] , [2] , [3] , [4] . Unintended cues generated by such non-signalling behaviours are thought to be modified to enhance their efficacy as communication signals through exaggeration of amplitudes, increases in regularity of rhythm and stereotypy, and changes in the relative timing of pattern elements [1] . Many informal hypotheses on signal origins are inferred exclusively from behavioural comparisons within or between species. For example, a cricket song, generated by rubbing wings together, is hypothesized to have evolved from inadvertent sound production associated with pheromone release [5] or movements associated with flight [6] . The peacock tail-fan display is thought to have originated from bowing and pecking at the ground to present food to females [7] . Formal testing of such hypotheses proves challenging, as it is necessary to conduct a phylogenetic comparison between species, and document homologous behaviours representing different stages of the ritualization process. The purpose of our study is to test the hypothesis that ritualized territorial signals in caterpillars that resolve conflicts using vibratory signals evolved from vibratory cues associated with locomotion. The masked birch caterpillar, Drepana arcuata (Walker) (Drepanidae: Drepaninae), communicates ownership of its territory using complex vibratory displays [8] . Resident caterpillars construct silken leaf shelters that they defend against intruding conspecifics by performing a repetitive vibratory display involving three principal elements: anal scraping, mandible drumming and mandible scraping ( Fig. 1 ). These caterpillars possess specialized structures on their anal segment that they drag across the leaf to make a scratching noise, which they produce while drumming or scraping their mandibles at varying rates to create a complex signal display. Consistent with other territorial displays in animals, these signals are generated primarily by the resident; they escalate in rate and kind as the encounter proceeds, and typically result in the intruder leaving the territory ( Supplementary Video 1 S1 ). This unusual form of communication in D. arcuata is highly ritualized, allowing both opponents to resolve contests without physical harm. 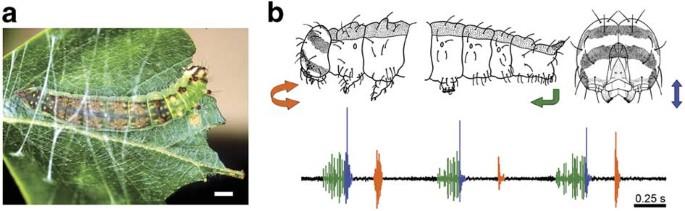Figure 1: Vibratory communication signals in the masked birch caterpillar,Drepana arcuata. (a) Caterpillars build and occupy silken leaf shelters (scale bar, 2.5 mm). (b) When approached by an intruder, the resident produces three types of vibratory signals: anal scraping (green) is performed by pulling the abdominal segment forward while at the same time scratching a sclerotized 'oar' against the leaf surface; mandible drumming (blue) and mandible scraping (orange) are produced by rapidly hitting and laterally scraping opened mandibles against the leaf surface, respectively. Figure 1: Vibratory communication signals in the masked birch caterpillar, Drepana arcuata . ( a ) Caterpillars build and occupy silken leaf shelters (scale bar, 2.5 mm). ( b ) When approached by an intruder, the resident produces three types of vibratory signals: anal scraping (green) is performed by pulling the abdominal segment forward while at the same time scratching a sclerotized 'oar' against the leaf surface; mandible drumming (blue) and mandible scraping (orange) are produced by rapidly hitting and laterally scraping opened mandibles against the leaf surface, respectively. Full size image In seeking hypotheses to explain the evolutionary origin of vibratory signalling, we performed a survey of literature that included preliminary morphological [9] , [10] or behavioural [11] , [12] descriptions of drepanid caterpillars. We observed a range of morphologies and behaviours associated with the anal segment across species. Most interestingly, it was noted that many species lacked anal prolegs, whereas others possessed a pair of fully functional prolegs. Prolegs are unsegmented legs located on abdominal segments 3–6 and 10 in most caterpillars [13] , [14] and are used for locomotion. This observation of morphological variation in the anal segment led to our hypothesis that the ritualized anal scraping signal seen in D. arcuata was co-opted from crawling. Specific predictions that would support this hypothesis include the following: (1) structures and movements in species that use their anal segment for crawling will be homologous to the modified forms found in anal scraping species; (2) the possession of anal prolegs will be the basal condition when mapped onto a phylogeny; and (3) anal scraping signals will possess modifications characteristic of ritualized signals when compared with cues associated with crawling. To test these predictions, we studied the morphological, behavioural and associated vibratory characteristics of the anal segment in distantly related species. We then constructed a molecular phylogeny onto which walking and talking with the anal segment were mapped. Comparative morphology of the anal segment Examinations of the terminal abdominal segment in 36 species of Drepanidae revealed interesting morphological diversity (see Methods and Table 1 ). Most notably, whereas some species possess fully formed anal prolegs, others lack these prolegs altogether ( Fig. 2 ). Furthermore, some species that lack anal prolegs possess a pair of specialized oar-shaped structures (anal oars) resembling thicker, hardened versions of small hairs (setae) commonly found on the surface of a caterpillar's body. The number and position of primary setae are relatively conserved throughout the order Lepidoptera and each primary seta is assigned a specific identity [13] , [14] . In 17 species of Drepanidae ( Table 1 ), detailed comparisons of the primary anal setae were made and homologues were identified. On the basis of the position and relative position of other known setae, we concluded that the anal oar is homologous to the posterior proctor seta or PP1 ( Fig. 2b,f ) that has undergone modification through sclerotization to become a stridulatory organ specialized for communication. Table 1 Lepidoptera specimens (ingroup taxa) and corresponding details of their morphology, behaviour and genes sequenced. 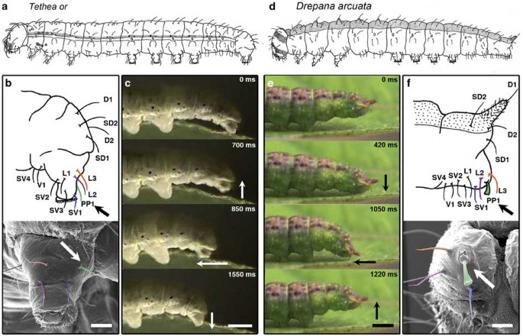Figure 2: Structure and function of the terminal abdominal segment in a representative species that possesses anal prolegs (Tethea or) and one that lacks anal prolegs but possesses anal oars (Drepana arcuata). (a,d) Schematic ofT. orandD. arcuataillustrating the overall body plan of each species. (b,f) (top panels) Schematic of identified setae on the terminal segment inT. orandD. arcuata; labels refer to names of setae according to Stehr13(D=dorsal, SD=subdorsal, V=ventral, SV=subventral, L=lateral, PP=posterior proctor); (bottom panels) scanning electron micrographs showing posterior views of the right anal proleg inT. orand the homologous region with stridulatory oar inD. arcuata. PP1 setae are marked with arrows, and colours correspond to setae labelled in the top panel. Scale bars, 200 μm (T. or) and 100 μm (D. arcuata). (c,e) Video frames of the terminal abdominal segments in each species, illustrating one complete crawling cycle inT. orand one complete anal scraping movement inD. arcuata. Arrows show the progression of movement. Scale bars, 3 mm (T. or) and 1.5 mm (D. arcuata). Full size table Figure 2: Structure and function of the terminal abdominal segment in a representative species that possesses anal prolegs ( Tethea or ) and one that lacks anal prolegs but possesses anal oars ( Drepana arcuata ). ( a , d ) Schematic of T. or and D. arcuata illustrating the overall body plan of each species. ( b , f ) (top panels) Schematic of identified setae on the terminal segment in T. or and D. arcuata ; labels refer to names of setae according to Stehr [13] (D=dorsal, SD=subdorsal, V=ventral, SV=subventral, L=lateral, PP=posterior proctor); (bottom panels) scanning electron micrographs showing posterior views of the right anal proleg in T. or and the homologous region with stridulatory oar in D. arcuata . PP1 setae are marked with arrows, and colours correspond to setae labelled in the top panel. Scale bars, 200 μm ( T. or ) and 100 μm ( D. arcuata ). ( c , e ) Video frames of the terminal abdominal segments in each species, illustrating one complete crawling cycle in T. or and one complete anal scraping movement in D. arcuata . Arrows show the progression of movement. Scale bars, 3 mm ( T. or ) and 1.5 mm ( D. arcuata ). Full size image Comparative behaviour of the anal segment Behavioural analysis of 13 Drepanidae species also revealed interesting differences in the use of the anal segment between morphological variants (see Table 1 ). Species that possess fully formed anal prolegs (including those belonging to Cyclidiinae and Thyatirinae) use them primarily during crawling, which is typical of most larvae in other lepidopteran families [14] . Crawling movements using the anal segment are illustrated in an exemplar species that possesses anal prolegs, Tethea or (Denis and Schiffermüller) (Drepanidae: Thyatirinae) ( Fig. 2a–c ; Supplementary Video S2 ). Forward locomotion involves a wave of longitudinal contractions that begins at the posterior end of the animal and travels towards the anterior end. The wave begins in the anal segment (A10) during a forward step of the anal prolegs. As the anal prolegs are planted ( Fig. 2c , frame 1), the wave moves through the body and the prolegs on segments A6–A3 are lifted and carried forward sequentially, causing the segments A7–A9 to be stretched. When the wave reaches the thoracic segments, the crochets on A10 that hold the anal proleg on the substrate are retracted, allowing the proleg to be lifted ( Fig. 2c , frame 2). As the next wave of contractions begins, the proleg is carried forward ( Fig. 2c , frame 3), the crochets are protracted and the prolegs grasp onto the substrate ( Fig. 2c , frame 4). Species that lack anal prolegs but possess anal oars, such as Drepaninae, use the anal segment for an entirely different purpose—to produce vibratory signals by anal scraping. This behavioural variant is described in the representative species, D. arcuata ( Fig. 2d–f ) ( Supplementary Video 3 S3 ). Before the anal scrape, the anal segment is slightly raised above the substrate and is placed parallel to the body ( Fig. 2e , frame 1). The anal scraping movement begins with a slight extension of the anal segment. The segment is then lowered and curled under so that the anal oars make contact with the leaf ( Fig. 2e , frame 2). The anal oars are dragged anteriorly across the leaf surface through a retraction of segments A7–A10 ( Fig. 2e , frame 3), and the anal segment is lifted off the substrate and re-extended to begin the next anal scrape ( Fig. 2e , frame 4). Although movements in the anal segments of these morphological conditions serve entirely different functions, their motor patterns seem to be homologous. Although the initial movements in anal scraping and crawling differ, the anal segments are similarly retracted into the sixth abdominal segment to scrape the anal oars on the leaf surface in D. arcuata and similar species ( Fig. 2e , frame 3), and to carry the anal proleg forward in T. or and similar species ( Fig. 2c , frame 3). On the basis of these observations, we conclude that the anal scraping movement is a modified component of crawling, and that instead of moving forward, D. arcuata walks on the spot, to talk. In addition to the two conditions described above (anal prolegs and crawling, and no anal prolegs and anal scraping), there is a third general morphological condition in some members of the Drepanidae species—ones that lack both anal prolegs and anal oars (see Fig. 3 ; Table 1 ). These species are peculiar as they do not use their anal segments for crawling or for sound production and the movements produced with this segment vary. Some species with this condition, such as Oreta rosea (Walker), have long processes emerging from the anal shield that they quickly sway from side to side when disturbed, perhaps to ward off a predator or parasitoid. Other species, such as Watsonalla cultraria (Fabricius), produce the same anal scraping movements as D. arcuata but produce no detectable vibration signals as they lack the modifications of anal oars. This morphological alternative could represent an intermediate condition, a secondary loss of prolegs, or a loss of anal oars. 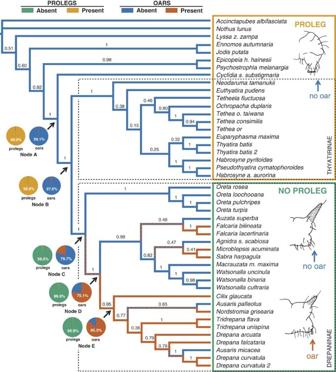Figure 3: Bayesian tree showing ancestral and derived states of the terminal (anal) segment. Anal prolegs present (orange), absent (green); anal oars present (red), absent (blue). Posterior probabilities are shown above branches. Pie charts are maximum likelihood probabilities of ancestral states at four selected nodes. The common ancestor of Drepaninae and Thyatirinae (Node B) had a 99.9% probability of possessing anal prolegs. Anal oars were probably gained at Node C and were subsequently lost multiple times. Figure 3: Bayesian tree showing ancestral and derived states of the terminal (anal) segment. Anal prolegs present (orange), absent (green); anal oars present (red), absent (blue). Posterior probabilities are shown above branches. Pie charts are maximum likelihood probabilities of ancestral states at four selected nodes. The common ancestor of Drepaninae and Thyatirinae (Node B) had a 99.9% probability of possessing anal prolegs. Anal oars were probably gained at Node C and were subsequently lost multiple times. Full size image Phylogeny of Drepanidae To assess the relationships among these morphological and corresponding behavioural variants in Drepanidae, we constructed a molecular phylogeny onto which the three morphological conditions were mapped ( Fig. 3 ). The phylogeny includes 36 ingroup ( Table 1 ) and 7 outgroup species ( Table 2 ), chosen on the basis of the availability of specimens and biological information. Outgroups were chosen following the composition of the superfamily according to Minet [15] . The tree was constructed from a concatenated data set of nuclear coding (CAD), nuclear ribosomal (28S D2) and mitochondrial (ND1) genes. Maximum likelihood probabilities for the presence/absence of anal prolegs and anal oars were calculated for five nodes on this tree with posterior probability of 1 (see Methods). Our results show that the presence of anal prolegs represents the ancestral condition in this group ( Fig. 3 ). The common ancestor of the clade constituting Drepaninae and Thyatirinae (Node B) had a 99.9% probability of possessing anal prolegs, which were subsequently lost in the monophyletic Drepaninae (Node C). Anal oars were likely to have been gained in the common ancestor at Node D or E, and were subsequently lost multiple times. Our results indicate that the two morphologies are not significantly correlated over phylogeny (lnL difference, 4.37; P =0.07; d.f.=4). Our phylogeny supports our hypothesis that anal oars (used for talking) are derived from ancestors that had anal prolegs (used for walking). Our results also show that the absence of oars in Drepanidae is due to several secondary losses, except in the case of the Oreta species, which may not have had oars in the first place. Table 2 Lepidoptera specimens (outgroup taxa), and corresponding details of their morphology and genes sequenced. Full size table Comparative territorial behaviour A comparative analysis of territorial behaviour provides insight into the contextual framework for the origin of anal signalling. Territorial behaviour was analysed in 13 Drepanidae species during conspecific encounters, and trends were observed within subfamilies ( Table 1 ). For example, Cyclidia substigmaria (Cyclidiinae), which possesses anal prolegs and lacks anal oars, does not exhibit territorial behaviours, and this seems to represent a common trend among other Cyclidiinae caterpillars (S.-H. Yen, personal observation). Thyatirinae caterpillars, on the other hand, which also possess anal prolegs, are highly territorial. Typically, encounters involve the resident using their anal prolegs to crawl towards the intruder, and either signal with mandibles or physically attack with the anterior segment (for example, pushing, hitting and biting). Drepaninae caterpillars, which lack anal prolegs, use mainly signalling to resolve conflicts. Encounters with Drepaninae species possessing anal oars typically involve anal scraping, followed by mandibular signalling. We hypothesize that anal scraping signals derive from locomotory movements associated with aggressive encounters in species lacking anal oars. To test this hypothesis, we examined in detail the behavioural patterns during territorial encounters in two representative species, T. or (Thyatirinae) and D. arcuata (Drepaninae) ( Fig. 4 ). T. or occupies and defends a leaf shelter comprising two leaves sewn together with silk ( Fig. 4a ; Supplementary Video 4 S4 ). In this species, a typical behavioural sequence begins with the resident crawling towards the intruder, followed by head movements including pushing (or biting; see Methods) and mandible scraping ( Fig. 4b,c left panel). Crawling towards the intruder is followed by pushing the intruder with the head (72.7% probability, z =9.60, P =<0.001, n =7), which is in turn followed by crawling (79.2%, z =6.18, P =<0.001, n =7). Occasionally, the caterpillar will follow the push with a mandible scrape (20.8%, z =−0.26, P =0.79, n =7), which is followed by a return to crawling (83.9%, z =5.21, P =<0.001, n =7). In D. arcuata , the resident begins an encounter with anal scraping followed by signalling with mandibles ( Fig. 4b,c right panel). Anal scraping is followed by mandible drumming (74.3%, z =17.0, P =<0.001, n =13), which is followed by another anal scrape (58.9%, z =5.53, P =<0.001, n =13). After a mandible drum, caterpillars will occasionally mandible scrape (32.5%, z =4.01, P =<0.001, n =13) before returning to an anal scrape (87.7%, z =10.9, P =<0.001, n =13). Physical aggression (biting, pushing and hitting) was never observed in D. arcuata trials. When comparing behavioural sequences between these two species ( Fig. 4c ; Supplementary Video S1, S4 ), our results indicate that anal scraping is derived from the intended motion of crawling towards a nest intruder, and that mandible signalling is derived from aggressive movements associated with anterior body parts, such as pushing, hitting and biting. Although more species need to be examined to resolve more clearly the evolutionary origins of different signalling elements, our results provide evidence that the ritualized signals of D. arcuata derive from aggressive non-signalling behaviours in more basal groups. We argue that cues associated with body movements previously associated with physical fighting became ritualized, permitting the resolution of a conflict without damage to either contestant. 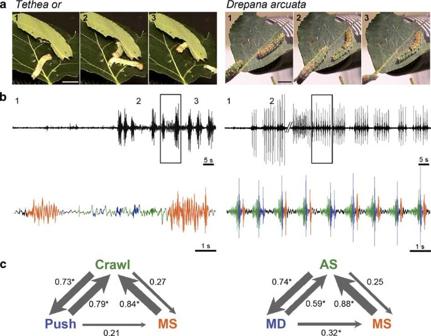Figure 4: Representative territorial encounters in a species that do not signal with their abdomen (Tethea or, left panel), and one that uses abdominal 'oars' to signal (Drepana arcuata, right panel). (a) Video frames illustrating a typical encounter between a resident and intruder, whereby the intruder enters the leaf shelter (1), the resident then approaches the intruder while hitting, pushing or mandible scraping (T. or; scale bar, 9 mm), or uses ritualized signals (D. arcuata; scale bar, 7 mm) (2) and the intruder turns to leave (3). (b) Laser vibrometer traces of the cues and signals on the leaf during such an encounter. Numbers correspond to frames ina. Relative amplitudes are equal between species. The box encloses part of the trace that is enlarged in the coloured segment below, which shows the vibrations generated by the resident when the two individuals are close together. Colours correspond to cues or signals inc. (c) Transition diagrams showing the probability of one type of behaviour following another. Asterisks denote significantly more probable transitions (D. arcuata,n=13;T. or,n=7;P<0.05). MS, mandible scraping; AS, anal scraping; MD, mandible drumming. Figure 4: Representative territorial encounters in a species that do not signal with their abdomen ( Tethea or , left panel), and one that uses abdominal 'oars' to signal ( Drepana arcuata , right panel). ( a ) Video frames illustrating a typical encounter between a resident and intruder, whereby the intruder enters the leaf shelter (1), the resident then approaches the intruder while hitting, pushing or mandible scraping ( T. or ; scale bar, 9 mm), or uses ritualized signals ( D. arcuata ; scale bar, 7 mm) (2) and the intruder turns to leave (3). ( b ) Laser vibrometer traces of the cues and signals on the leaf during such an encounter. Numbers correspond to frames in a . Relative amplitudes are equal between species. The box encloses part of the trace that is enlarged in the coloured segment below, which shows the vibrations generated by the resident when the two individuals are close together. Colours correspond to cues or signals in c . ( c ) Transition diagrams showing the probability of one type of behaviour following another. Asterisks denote significantly more probable transitions ( D. arcuata , n =13; T. or , n =7; P <0.05). MS, mandible scraping; AS, anal scraping; MD, mandible drumming. Full size image The evolution of a novel communication signal must necessarily co-evolve with receiver detection. Thus, vibration cues associated with non-signalling movements in 'ancestral' behaviours must be available to the receiver. Moreover, communication theory holds that during the process of ritualization, such inadvertent cues undergo specific modifications that render them more accessible and less ambiguous to the receiver: (1) simplification (reduction of the number of components); (2) exaggeration (increased amplitude of remaining components); (3) repetition (increased repetition rates of remaining components); and (4) stereotypy (reduction in the variance of the cue) [1] . Using a laser vibrometer, we recorded vibrations on the leaf produced during conspecific interactions in 11 species (see Table 1 ). Detailed comparisons of these vibratory recordings were made in two representative species, D. arcuata and T. or , to determine whether cues were associated with non-signalling movements (that is, crawling and pushing) and to compare these cues with ritualized signals (see Methods). Figure 4b (left panel) shows that non-signalling territorial behaviours (crawling and pushing) in T. or generate vibration cues detectable by our laser vibrometer above the background noise. On comparing body movements associated with anal scraping ( D. arcuata ) and crawling ( T. or ), we found that anal scraping has fewer body movements (simplification; five components using four body segments in anal scraping versus 17 components using 10 body segments for crawling) and produces vibrations of significantly larger amplitude (exaggeration; t =5.04, P <0.001, d.f.=10, paired t -test) that are repeated at a significantly higher rate (repetition; t =−3.68, P =0.0024, d.f.=14.07, t -test). Increased stereotypy is also clearly evident by more regularity in the periodicity, amplitude and signal sequences produced by D. arcuata residents in comparison with T. or ( Fig. 4b ). These results provide further support for our hypothesis that vibratory cues associated with crawling towards the intruder become ritualized into a communication signal. In summary, our results support our hypothesis that a ritualized territorial signal—anal scraping—is derived from a locomotory pattern—crawling—observed in ancestral species. Moreover, we provide evidence for the contextual framework of signal evolution by showing that other signalling components—mandible drumming and scraping—became substitutes for more physically aggressive behaviours such as pushing, hitting and biting. Thus, several evolutionarily derived species within this group use a 'civilized' alternative to physical fighting. Many other animals resolve conflicts using ritualized displays thought to derive from behaviours associated with physical aggression. Foot drumming in kangaroo rats [16] and pawing the ground in bulls are thought to have evolved from intentions to chase, and human sports events such as the Olympic games are suggested to represent ritualized fighting displays [17] . However, the evolutionary pathways leading to such ritualized displays remain untested. Our study provides direct experimental evidence for the evolutionary origin of a communication signal, and supports the fundamental tenets of ritualization suggested by classic ethologists. Further research on this unique model system of vibratory caterpillars should examine the environmental selection pressures that influenced ritualization, as well as the changes to the neuromuscular system accompanying the transition from walking to talking. Animals Living and preserved larvae used in this study were obtained from various sources (see Table 1 ). Larvae were reared indoors on cuttings of their respective host plants under a light–dark (18:6) photoperiod at 21–26 °C. All larvae used for experiments were late instars (third to fifth) occupying solitary leaves or leaf shelters, with the exception of Cyclidia substigmaria substigmaria (Cyclidiinae), which live gregariously. Morphology We examined the anal segments (A8–A10) of larvae preserved in 80% ethyl alcohol. Drawings were made using a drawing tube and setae were identified and labelled following the nomenclature described by Stehr [13] and I. Hasenfuss (personal communication). For scanning electron micrographs, anal segments were air dried or prepared in HMDS (hexamethyldisilazane) [18] . Specimens were sputter coated with gold palladium and examined using a JEOL scanning electron microscope (JSM-6400; JEOL). Morphological characteristics of the anal segment in some species were obtained from literature, as indicated in Table 1 . Phylogenetic analysis Total genomic DNA was extracted from 43 adult moths (see Tables 1 and 2 ) stored in 100% ethyl alcohol at −80 °C. A single leg from each sample was ground and then digested at 58 °C for 1 h with 20 mg ml −1 proteinase K in 250 μl of a solution containing 0.1 M Tris (pH 8.0), 10 mM EDTA and 2% SDS. Samples were then incubated at 65 °C for an additional 10 min in a solution containing 5 M NaCl and 10% cetyl trimethylammonium bromide. The solutions were extracted using standard phenol–chloroform protocols and DNA was precipitated overnight in 95% ethyl alcohol. DNA fragments were amplified by PCR using specific primers for three genes—CAD, ND1 and 28S D2. Amplifications were carried out in 20 μl volumes containing 3 μl of each primer, 2.0 μl of 10× Taq buffer containing MgCl 2 (Bioshop), 1.2 μl MgCl 2 (Bioshop), 0.4 μl of an equimolar solution of dNTPs (Invitrogen), 0.5 μl of Taq polymerase (Bioshop), 7.9 μl dH 2 O and 2 μl DNA template. A typical PCR procedure for all genes consisted of 3 min denaturation at 95 °C, followed by 30 cycles including denaturation (30 s at 95 °C), annealing (30 s, temperatures are given below) and extension (30 s at 72 °C). An additional 10 min extension step at 72 °C was included in the final cycle. PCR products were verified by agarose gel electrophoresis and either purified using a GenElute PCR Clean-Up Kit (Sigma-Aldrich) for direct sequencing or cloned using a TOPO Cloning Kit (Invitrogen) before sequencing multiple clones of each fragment. The second expansion segment of the 28S gene was amplified using primers 28S D2F: 5′-AGAGAGAGTTCAAGAGTACGTG-3′ and 28S D2R: 5′-TTGGTCCGTGTTTCAAGACGGG-3′ (ref. 19 ) at an annealing temperature of 59 °C. An 849 bp region of the CAD gene was amplified using primers 743nF: 5′-GGNGTNACNACNGCNTGYTTYGARCC-3′ and 1028R: 5′-TTRTTNGGNARYTGNCCNCCCAT-3′ (ref. 20 ) at an annealing temperature of 50 °C. Often it was necessary to follow this amplification with a second amplification using nested primers at 50 °C (791F: 5′-TTYGARGARGCNTTYCARAARGC-3′ and 963R: 5′-GCRCACCARTCRAAYTC-3′ (ref. 20 )). For ND1, we designed Drepanidae-specific primer pairs based on Weller et al . (ref. 21 ) 5′-GAGCCAGGTTGGTTTCTATC-3′ and 5′-GAATTAGAAGATCAACCAGCAA-3′, and used an annealing temperature of 53 °C. Both strands of gel-purified or cloned DNA fragments were sequenced in an Applied Biosystems 3730 DNA Analyzer (Applied Biosystems). Sequence contigs were viewed, assembled and edited using DNA Baser (HeracleSoftware). Sequences were aligned in MAFFT [22] using an E-INS-I setting with 1,000 iterations, and also checked by eye. The optimal nucleotide substitution model for each gene was determined with the Akaike Information Criterion [23] , as implemented in Modeltest [24] . The best-fit models were GTR+G (28S) and GTR+I+G (CAD, ND1). The data sets were concatenated into a single data set of 1,617 base pairs, including 680 informative sites (CAD—638 base pairs, 242 informative sites; ND1—450 base pairs, 190 informative sites; and 28S D2—529 base pairs, 248 informative sites) and the appropriate substitution model partitioned for each gene. Phylogenetic analysis was conducted in MrBayes [25] with eight chains, sampling every 1,000 generations with a heating temperature parameter of 0.12. The Markov chain was terminated at 25 million generations, determined by examining trace plots in AWTY [26] . We coded anal prolegs and oars as discrete binary presence/absence characters in Mesquite [27] . We inferred ancestral conditions of anal prolegs and oars for four selected nodes, with posterior probability of 1 in Mesquite using the Mkv model for morphological character data [28] . We used Bayes traits [29] to determine whether the two traits were strongly correlated on phylogeny following the method outlined by Pagel [30] . The fully aligned, concatenated data matrix can be accessed as a Supplementary file ( Supplementary Data S1 ). Behavioural analyses and vibration recordings Behaviours associated with the anal segment, territorial interactions and vibratory signals and cues were studied directly in 11 species representing all three subfamilies. In addition, behavioural characters for two species were obtained through personal communication from I. Hasenfuss. A full list of species and behavioural characters obtained is provided in Table 1 . Detailed comparisons of behaviours and signals associated with territorial encounters were performed on two species, T. or and D. arcuata , which represented Thyatirinae and Drepaninae, respectively. Territorial behaviours were not scored for the other sister group, Cyclidiinae, as the representative species for this group did not exhibit territorial behaviour. To compare territorial behaviour patterns and associated vibratory signals and cues between D. arcuata and T. or , we staged within-species encounters between a resident larva and an introduced intruder of approximately the same size, and then compared the results between species. All trials were videotaped with a digital camcorder and a remote audio microphone placed 1–2 cm behind the leaf, or with a laser Doppler vibrometer. Residents were placed on a leaf of their respective host plants and left undisturbed for at least 60 min. Before the trial, intruders were isolated in a container with bare twigs for 15–20 min. Intruders were then placed on the petiole of the leaf and resident behaviours were observed from the time the intruder entered the leaf shelter to when it left. After the trial, both caterpillars were isolated in a separate container so that they would not be used in another trial. Behaviours were scored from 13 D. arcuata encounters and 7 T. or encounters using a computerized event recorder [31] . Such behavioural events included forward and backward crawling (each step counted as a separate event), turning 180° to face the intruder, remaining motionless or 'freezing', sitting in an 'S' position, feeding, mandible drumming, mandible scraping, anal scraping, making contact with the intruder using either the head or caudal end, pushing, laying silk and constructing a leaf shelter. Although biting was observed in T. or (our own observations and those of I. Hasenfuss), we did not score this behaviour, as it was difficult to distinguish between pushing and biting during our video analysis trials that typically took place with T. or larvae interacting within leaf shelters. Discrete time sequential analysis was performed to quantify frequency and transition probabilities between behaviours [31] (with accompanying z -scores and P -values). Transition diagrams ( Fig. 4 ) were created using only transition probabilities of 0.10 or higher. Vibrations measured using a Polytec Laser Doppler Vibrometer (PDV 100; Polytec) were digitized and recorded onto a Marantz Professional portable solid-state recorder (PMD 671; 44.1 kHz sampling rate; Marantz). Vibrations on the leaf surface were measured at the location of a circular piece of reflective tape (2.0 mm in diameter) positioned 1–2.5 cm from the resident caterpillar. All vibration recordings were made in an acoustic chamber (Eckel Industries) in conjunction with video recording. Oscillograms were produced using the Raven Bioacoustics Research Program (Cornell Laboratory of Ornithology). To determine whether the vibrational signals of D. arcuata met the four main conditions for ritualization, the signals were compared with crawling patterns in T. or on the basis of simplification, exaggeration, repetition and stereotypy. To quantitatively compare the simplicity of movements between species, components of each behaviour were counted and compared directly, wherein each component comprised a single directional change in movement. Exaggeration was assessed by comparing the relative amplitude of vibration signals associated with crawling and anal scraping within given trials of D. arcuata . Because of differences in leaf structure and size of the individuals between trials, amplitudes of D. arcuata anal scraping could not be compared directly with crawling in T. or . However, it was found that vibrations produced by crawling were comparable between species, and therefore anal scraping in resident D. arcuata caterpillars was compared with intruder crawling within the same trials using a paired t -test. Amplitude measurements were taken for 11 trials using the Raven Bioacoustics Research Program and behaviours were compared. Repetition was assessed by comparing rates of anal scraping in D. arcuata with rates of crawling in T. or within the 20 s period following the time of closest contact. Rates were compared between 16 individuals of D. arcuata and 9 individuals of T. or using a t -test. All statistical tests were performed with a 95% confidence interval. Data deposition . All sequences were submitted to GenBank under accession numbers GU174157 , GU174263 . How to cite this article: Scott, J.L. et al . The evolutionary origins of ritualized acoustic signals in caterpillars. Nat. Commun. 1:4 doi: 10.1038/ncomms1002 (2010). Copyright: © 2010 Scott, J.L. et al. This is an open-access article distributed under the terms of the Creative Commons Attribution License, which permits unrestricted use, distribution, and reproduction in any medium, provided the original author and source are credited.